Programmable energy landscapes for kinetic control of DNA strand displacement DNA is used to construct synthetic systems that sense, actuate, move and compute. The operation of many dynamic DNA devices depends on toehold-mediated strand displacement, by which one DNA strand displaces another from a duplex. Kinetic control of strand displacement is particularly important in autonomous molecular machinery and molecular computation, in which non-equilibrium systems are controlled through rates of competing processes. Here, we introduce a new method based on the creation of mismatched base pairs as kinetic barriers to strand displacement. Reaction rate constants can be tuned across three orders of magnitude by altering the position of such a defect without significantly changing the stabilities of reactants or products. By modelling reaction free-energy landscapes, we explore the mechanistic basis of this control mechanism. We also demonstrate that oxDNA, a coarse-grained model of DNA, is capable of accurately predicting and explaining the impact of mismatches on displacement kinetics. As a result of its predictable and controllable binding interactions, DNA is an adaptable material for nanoscale self-assembly [1] , [2] , [3] , [4] , [5] , [6] . DNA hybridization, programmed through design of base sequence, allows facile production of functional nanostructures such as synthetic membrane pores [7] , plasmonic devices [8] and calibration standards for super-resolution microscopy [9] . It can also be used to create dynamic nanodevices such as guidable robots [10] , [11] , [12] , [13] and molecular actuators [14] , as well as chemical reaction networks capable of performing neural network computation [15] or matrix multiplication [16] . One of the most fundamental reactions underlying virtually all such dynamic DNA systems is toehold-mediated strand displacement [17] , [18] , a process in which one strand of a duplex is replaced by another to create a more stable complex ( Fig. 1 ). The thermodynamic preference for the invading strand is provided by the toehold, a domain of the target strand that is initially single-stranded and to which the invader can bind to initiate the reaction. 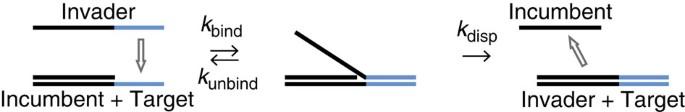Figure 1: Toehold-mediated strand displacement. An incumbent strand is initially hybridized to a complementary ‘displacement’ domain (black) of a target strand by Watson-Crick base pairing. The invader strand is complementary both to the displacement domain of the target and to an adjacent ‘toehold’ domain (blue), allowing it to displace the incumbent to form a more stable duplex. Displacement can be initiated by binding of the invader to the toehold followed by a branch migration process in which base pairs between target and incumbent break and are replaced by base pairs with the invader. The overall reaction rate for strand displacement is strongly dependent on the toehold binding strength17,18,19. Figure 1: Toehold-mediated strand displacement. An incumbent strand is initially hybridized to a complementary ‘displacement’ domain (black) of a target strand by Watson-Crick base pairing. The invader strand is complementary both to the displacement domain of the target and to an adjacent ‘toehold’ domain (blue), allowing it to displace the incumbent to form a more stable duplex. Displacement can be initiated by binding of the invader to the toehold followed by a branch migration process in which base pairs between target and incumbent break and are replaced by base pairs with the invader. The overall reaction rate for strand displacement is strongly dependent on the toehold binding strength [17] , [18] , [19] . Full size image In the dominant reaction mechanism, toehold-mediated strand displacement is initiated by binding of the invader to the toehold. The invader then replaces the incumbent bases, one by one, by branch migration, a random walk of the branch point between the domain of the target that is hybridized to the invader and that still hybridized to the incumbent [17] , [18] , [19] . If the branch point advances sufficiently far that the incumbent is completely displaced then the strand-exchange reaction is complete. However, when the branch point returns to the beginning of the displacement domain the invader does not necessarily dissociate: it may remain bound to the toehold and re-initiate displacement of the incumbent. The probability that the incumbent is successfully displaced, and hence the overall reaction rate, is thus strongly dependent on toehold stability. For sufficiently dilute systems, strand exchange can be approximated as a second-order reaction. By changing the sequence and length of the toehold, and thus the free energy of toehold binding, the second-order reaction rate constant can be adjusted between 1 and 10 7 M −1 s −1 (refs 17 , 18 ). Variants of the system have been explored to increase control over this process. Examples include the introduction of an inert spacer between toehold and displacement domains [20] and the introduction of mismatches (non-Watson-Crick base pairs) between the invader and the target [21] , [22] , [23] , [24] , [25] , [26] , [27] , [28] . In general, these schemes couple a change in the reaction rate constant to a change in the free-energy gain associated with the strand-displacement reaction. Here, we introduce a mechanism for kinetic control of strand displacement that decouples changes in the reaction rate from changes in the standard free energy of the reaction. By altering the position of a sequence mismatch created by an invader within the displacement domain, the reaction rate constant can be tuned over three orders of magnitude without significantly affecting the free-energy change. Detailed modelling of the sequence of reaction intermediates, using a coarse-grained DNA model [29] , [30] that accurately predicts relative reaction rate as a function of mismatch location, allows us to propose a detailed model of the reaction pathways. We demonstrate the application of this tool for kinetic control to create a competitive strand-displacement system in which the most rapidly formed product is transient and is replaced by a more stable complex. Kinetic control through position of a mismatch To investigate the effects of a single mismatch between the invading strand and target on a toehold-mediated strand-displacement process ( Fig. 2 ), we use an indirect reporter system [18] in which the displaced incumbent strand in turn displaces a fluorescently labelled strand from a reporter duplex ( Fig. 2b ). Emission from the Cy5 fluorophore is initially quenched by an IowaBlack® RQ quencher attached to the complementary strand of the reporter duplex. The increase in fluorescence when fluorophore and quencher are separated is used as a measure of the progression of the primary reaction. Use of a secondary reporter avoids the need for fluorescent labelling of the primary reactants, which might perturb their interaction [31] , [32] . Reactions with different mismatch positions and toehold lengths can be followed using a single reporter complex. This cascaded reaction system also serves as an initial demonstration that components controlled by mismatches can be incorporated into more complex reaction networks. 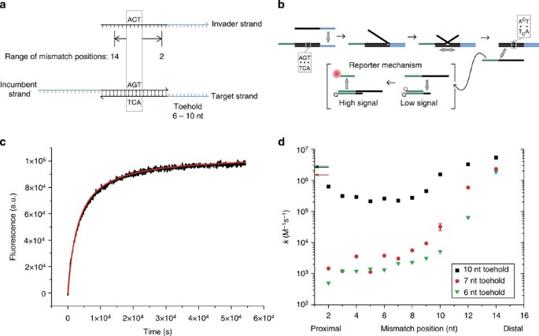Figure 2: Use of mismatched sequences to control strand-displacement kinetics. (a) An invader strand is able to displace an incumbent strand from a target strand with the help of a 6–10-nucleotide (nt) toehold. In doing so, the invader forms a C–C mismatch whose position within the invader–target duplex can be varied. Mismatch positionxrefers to a system where the mismatch is formedxnt from the toehold. The entire displacement domain over which the invader and incumbent compete is 17 nt long. (b) Displacement of the incumbent strand triggers the reporter mechanism, in which a fluorescent strand is released from a reporter duplex in which it was quenched. (c) The resulting fluorescence response (black) is fitted assuming second-order kinetics. These data correspond to an invading strand with a 6-nt toehold that creates a C–C mismatch 12 nt from the toehold. (d) Second-order reaction rate constants for strand displacement (k) measured for invading strands with different toehold lengths and mismatch positions. Arrows indicate the corresponding rate constants for ‘perfect’ invaders (that create no mismatches) with the same toeholds. In theSupplementary Information(Supplementary Note 1;Supplementary Figs 1 and 2;Supplementary Table 1), we discuss the use of a second-order rate constant to parameterize the data: for 6- and 7-nt toeholds this is a good approximation; for 10-nt toeholds with proximal and central mismatches there are systematic deviations from second-order kinetics, but the fitted rate constant quantifies the overall reaction speed in a manner that allows useful comparison with other systems. Statistical error on a single measurement was estimated to be ±22% by performing one displacement reaction tenfold (Supplementary Note 2). Figure 2: Use of mismatched sequences to control strand-displacement kinetics. ( a ) An invader strand is able to displace an incumbent strand from a target strand with the help of a 6–10-nucleotide (nt) toehold. In doing so, the invader forms a C–C mismatch whose position within the invader–target duplex can be varied. Mismatch position x refers to a system where the mismatch is formed x nt from the toehold. The entire displacement domain over which the invader and incumbent compete is 17 nt long. ( b ) Displacement of the incumbent strand triggers the reporter mechanism, in which a fluorescent strand is released from a reporter duplex in which it was quenched. ( c ) The resulting fluorescence response (black) is fitted assuming second-order kinetics. These data correspond to an invading strand with a 6-nt toehold that creates a C–C mismatch 12 nt from the toehold. ( d ) Second-order reaction rate constants for strand displacement ( k ) measured for invading strands with different toehold lengths and mismatch positions. Arrows indicate the corresponding rate constants for ‘perfect’ invaders (that create no mismatches) with the same toeholds. In the Supplementary Information ( Supplementary Note 1 ; Supplementary Figs 1 and 2 ; Supplementary Table 1 ), we discuss the use of a second-order rate constant to parameterize the data: for 6- and 7-nt toeholds this is a good approximation; for 10-nt toeholds with proximal and central mismatches there are systematic deviations from second-order kinetics, but the fitted rate constant quantifies the overall reaction speed in a manner that allows useful comparison with other systems. Statistical error on a single measurement was estimated to be ±22% by performing one displacement reaction tenfold ( Supplementary Note 2 ). Full size image Figure 2d shows how the rate constant for strand displacement depends on the position of a single mismatch within a 17-nt displacement domain. Three different toehold lengths and 11 different positions of the mismatch within the target displacement domain were tested. The reaction rate constant varies by up to three orders of magnitude depending on the position of the mismatch between the invader and target. Generally, a mismatch closer to the toehold (proximal mismatch) is a much greater impediment to strand displacement than the same mismatch at the end of the displacement domain (distal mismatch). Three different kinetic regimes are observed: a high-rate regime for distal mismatches; a low-rate regime for proximal mismatches; and a transition region in which the rate constant is strongly dependent on the mismatch position. Taking the 6-nt toehold as an example, we see a strong suppression of the reaction rate for mismatch positions ≤10, and almost no suppression with the mismatch at position 14. The difference in rate constant between proximal and distal mismatch positions is considerably more pronounced for shorter toeholds, despite the fact that for all toeholds used here the corresponding perfectly complementary invaders displace the incumbent strand with almost equal rates. The overall free-energy change of reaction, , quantifies the thermodynamic driving force associated with displacement. Differences in between systems are small and do not correlate with the observed systematic dependence of rates on mismatch position. NUPACK [33] estimates that lies in the range 3.1–4.2 kcal mol −1 for all displacement reactions with 7-nt toeholds reported in Fig. 2d : a change of 1.1 kcal mol −1 in the height of a simple activation barrier would only explain a change in reaction rate by a factor exp(1.1 kcal mol −1 /RT)<10. We see that the wide tunability of the strand-displacement rate through adjustment of the position of the mismatch created does not require significant changes in reaction free energy. Exploring strand displacement through energy landscapes A simple model for displacement is illustrated in Fig. 1 . Here we consider only three states: with no interaction between the invader and incumbent–target duplex; with the invader bound to the toehold; and after displacement. When introducing a mismatch that destabilizes the invader–target complex by ΔΔ G o , we would naively expect to create an activation barrier for displacement that would cause a reduction in the overall reaction rate of exp(−ΔΔ G o /RT) for weak toeholds (for which there is a high probability of transient toehold binding that does not lead to displacement), and almost no effect for strong ones (for which toehold binding is effectively irreversible). As single-base-pair mismatches are known to destabilize duplexes by ΔΔ G o ≈2–6 kcal mol −1 (ref. 34 ), a barrier that would give a rate reduction of two to four orders of magnitude, this model can account for the strongly reduced rate constants observed for invaders that create proximal mismatches. It does not, however, explain why the effect of the mismatch is so strongly dependent on its location. The reason for this failure is the limited resolution of the model: the branch migration process by which the invader displaces the incumbent is far too complex to be represented by a single reaction step. To overcome this deficiency in the model we use oxDNA, a recently developed coarse-grained DNA model [29] , [30] ( Supplementary Note 3 ; Supplementary Figs 3 and 4 ), which can be used to simulate the steps involved in strand displacement at a single-nucleotide level. Previously, oxDNA has been shown to give a good representation of strand displacement where base sequences are perfectly matched [19] . Simulations of displacement reactions with a 5-nt toehold and 16-nt displacement domain were used to calculate relative displacement rate constants for a perfectly matched invader and for invaders creating mismatches. These were compared with experimentally determined rate constants for the same systems. Results for perfect invader and invaders creating distal, central and proximal defects, respectively, are: experiment 1:0.4:0.008:0.001 and oxDNA simulation 1:0.6:0.009:0.003 ( Supplementary Note 3 ; Supplementary Tables 2–4 ). Although there is uncertainty associated with these simulation results (as described in the Methods section), oxDNA, which was parameterized using completely unrelated data [19] , [29] , predicts the observed dependence of displacement rate on mismatch position at a near-quantitative level. Most importantly, oxDNA captures the trend that distal mismatches have a relatively small effect on the reaction rate. The single-nucleotide resolution of oxDNA also provides a better qualitative understanding of the mismatch displacement process. 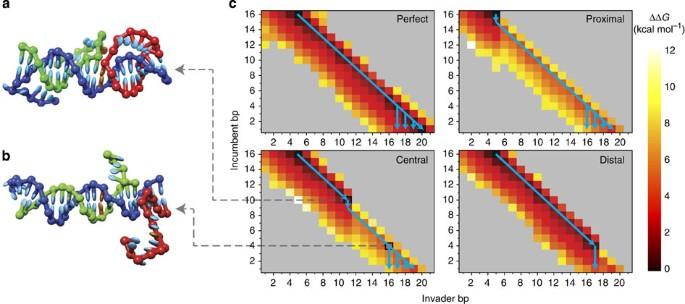Figure 3: Results of simulations of toehold-mediated strand displacement in which a mismatch is created in the invader–target duplex (5-nt toehold, 16-nt displacement domain). (a,b) representative simulation snapshots for an invader with a central mismatch. Ina, the invader (green) is bound to the target (blue) up to the mismatch site (gold). The incumbent (red) still occupies the later bases. Inb, the invader has overcome the mismatch and the incumbent is only bound to the target through four remaining base pairs. (c) Free-energy landscapes for four different invading strands: perfect invader, invaders creating proximal, central and distal mismatches. The coordinates are the numbers of base pairs formed between target and incumbent and between target and invader. The free energy of a state with the invader bound to the toehold but with no displacement (invader base pairs=5, incumbent base pairs=16) is set to zero. State (5,16) represents complete toehold binding without displacement of the incumbent. Grey states are unsampled. Blue arrows indicate representative reaction pathways from toehold initiation to displacement. Most states with low free-energy have a total of 21 base pairs, or 20 after the mismatch is formed. States in which not all target bases are paired are located towards the bottom left of each landscape; they correspond to spontaneous base melting/fraying. States in which the total number of base pairs exceeds the number of target bases are located towards the top right of each landscape and arise because the algorithm that counts paired bases can identify a target base as simultaneously paired with both incumbent and invading bases in some intermediate microstates. Figure 3 shows calculated free-energy landscapes during strand displacement. For the case of a perfectly complementary invader, the free-energy landscape reiterates what is already known about toehold-mediated strand displacement [18] , [19] . After toehold initiation, the invading strand can displace the incumbent through branch migration, as indicated by the blue arrow. Full displacement is not guaranteed every time toeholds bind, however, as the toehold can spontaneously detach before branch migration is initiated. Even if several steps of branch migration occur, the system can still return to a ‘toehold-only’ state and subsequently detach without displacing the incumbent. The stronger the toehold, the less likely it is that the invader will detach from the toehold-only state, however, which explains the strong dependence of displacement rate on toehold length previously observed [17] , [18] . Note that the energy landscape contains accessible, although energetically less-favourable, states adjacent to those where all bases of the target are paired with those from either incumbent or invader. These correspond to fraying of the duplexes, that is, spontaneous melting of one or more base pairs. If branch migration has progressed close to the end of the displacement domain, fraying of the few incumbent–target base pairs remaining can lead to complete detachment of the incumbent and thus provides a shortcut to successful displacement (vertical arrows near the bottom of each landscape in Fig. 3c ). Our simulations show that spontaneous melting of the last few base pairs plays a significant role in strand displacement: it is rare for the invader to have formed all but the final base pair at the moment when the incumbent detaches. In cases where branch migration has progressed 75% along the displacement domain from the toehold, for example, the probability for directly proceeding to full displacement before returning to a toehold-only state is 83%, instead of the 75% expected under the assumption that branch migration is an unbiased random walk process and provides the only pathway to full displacement. Figure 3: Results of simulations of toehold-mediated strand displacement in which a mismatch is created in the invader–target duplex (5-nt toehold, 16-nt displacement domain). ( a , b ) representative simulation snapshots for an invader with a central mismatch. In a , the invader (green) is bound to the target (blue) up to the mismatch site (gold). The incumbent (red) still occupies the later bases. In b , the invader has overcome the mismatch and the incumbent is only bound to the target through four remaining base pairs. ( c ) Free-energy landscapes for four different invading strands: perfect invader, invaders creating proximal, central and distal mismatches. The coordinates are the numbers of base pairs formed between target and incumbent and between target and invader. The free energy of a state with the invader bound to the toehold but with no displacement (invader base pairs=5, incumbent base pairs=16) is set to zero. State (5,16) represents complete toehold binding without displacement of the incumbent. Grey states are unsampled. Blue arrows indicate representative reaction pathways from toehold initiation to displacement. Most states with low free-energy have a total of 21 base pairs, or 20 after the mismatch is formed. States in which not all target bases are paired are located towards the bottom left of each landscape; they correspond to spontaneous base melting/fraying. States in which the total number of base pairs exceeds the number of target bases are located towards the top right of each landscape and arise because the algorithm that counts paired bases can identify a target base as simultaneously paired with both incumbent and invading bases in some intermediate microstates. Full size image The introduction of a mismatch adjacent to the toehold alters the energy landscape markedly ( Fig. 3c , ‘Proximal’). Once the toehold is bound, the system must enter an energetically less-favourable state to begin branch migration as the invader must immediately enclose a mismatch. This destabilizes the system by reducing the total number of base pairs formed, indicated by the short vertical arrow at the top of the displacement path. Since the rate of this transition is relatively low, the system is forced to spend considerably more time in the toehold-only state, creating a higher probability for spontaneous detachment of the invader and thus reducing the overall reaction rate. Since the toehold-detachment rate is dependent on toehold strength, the overall strand-displacement rate is also toehold dependent, as seen in Fig. 2 . Note that, even if the invader manages to overcome the mismatch, the ensuing random walk of the branch point is more likely to return the system to the toehold-only state than it is to result in full incumbent displacement. Moving the same mismatch to the centre of the displacement domain yields the ‘Central’ energy landscape in Fig. 3c . Although the energy barrier that the invading strand must overcome at the position of the mismatch remains virtually the same as in the proximal mismatch case, there are two distinct differences. First, the number of relatively easily accessible pre-mismatch states is increased: in addition to the toehold-only states there are now states in which the incumbent is partially displaced (5< incumbent base pairs <12). This reservoir of additional states stabilizes the invader/target duplex before enclosure of the mismatch. Once the mismatch has been enclosed, the distance to the end of the displacement domain is shorter, increasing the probability of successful displacement before the system falls back into a pre-mismatch state. These effects are reflected in the data in Fig. 2d : the rate constants for invaders with 6-nt and 7-nt toeholds are slightly higher for central mismatches than for proximal ones. Note that this effect is not significant for the 10-nt toehold systems for which there is a low probability of toehold dissociation. The similarity between the energy landscapes for a distal mismatch and for the perfect invader is striking. With the exception of states in which the invader forms >17 base pairs with the target (very close to full displacement of the incumbent), we can assume that the displacement process is the same. Once branch migration reaches a pre-mismatch state close to the end, the displacement ‘shortcut’ described above in the context of the perfect invader now allows completion of displacement before the invader encloses the mismatch. Our simulations of the distal mismatch system reveal that in 80% of cases detachment of the incumbent occurs without the invader having formed any contacts beyond the mismatch ( Supplementary Table 5 ). As negotiation of the energy barrier posed by the mismatch is not necessary for successful displacement, the impeding effect of a distal mismatch is very limited. Hence, the rate constants for distal mismatches are close to those for perfect invaders. The most stable state for all systems is a fully bonded invader–target duplex. Thus, distal mismatches are eventually enclosed, but only after dissociation of the incumbent, when displacement has already succeeded. The rate of spontaneous detachment of all incumbent bases beyond the mismatch is exponentially suppressed by the length of the duplex that must detach. This explains the sharp drop in displacement rates as the mismatch location is moved towards the toehold. The landscapes show that the free energy of the system is approximately independent of mismatch position after mismatch enclosure, and for strand displacement is approximately equal for all mismatch locations. This supports our claim that the effect of mismatch location on reaction rate is fundamentally a kinetic phenomenon rather than an equilibrium thermodynamic property. Using an elongated displacement domain We have also measured displacement rates for a system with a displacement domain of 25 nt instead of 17 nt. The two systems behave very similarly when the distance between the mismatch and the distal end of the displacement domain is the same ( Supplementary Note 4 ; Supplementary Fig. 5 ). This is consistent with our hypothesis that the relative ineffectiveness of a distal mismatch in reducing the strand-displacement rate is a result of spontaneous dissociation of the incumbent before creation of the mismatch. Branch migration up to the position of the mismatch is relatively insensitive to the number of base pairs before the mismatch [18] , [19] , whereas the rate of spontaneous melting of the last section of the duplex depends exponentially on the number of base pairs after the mismatch that must dissociate. The length of the displacement domain that must be traversed before detachment therefore contributes only weakly to the displacement rate; the length that must spontaneously detach is far more important. Fine-tuning rates with different types of mismatches From our qualitative exploration of the free-energy landscape for strand displacement, we deduce that an energetically more-favourable mismatch—and thus a lower energy barrier between pre- and post-mismatch states—has a lesser impact on reaction kinetics. This is consistent with the results of experiments with invading strands that form a instead of a mismatch ( Supplementary Note 5 ; Supplementary Figs 6 and 7 ). This suggests that the reaction rate constant of a specific displacement reaction could be fine-tuned by using different mismatches. Creating complex kinetic behaviour using mismatches The correlation between mismatch position and displacement rate constant can also be used to create more complex kinetic behaviours. As proof of principle, we designed a simple system in which two invading strands compete for the same displacement domain while relying on toeholds at opposite ends of the duplex to initiate the displacement reaction. By introducing a mismatch that is created by both invading strands, but is asymmetrically placed, one invader is kinetically favoured. By allowing the other invader to form additional base pairs, it is thermodynamically favoured. The system behaves as designed ( Fig. 4 ): the kinetically favoured invader dominates target binding early in the experiment but is replaced by the thermodynamically favoured strand as the system equilibrates. In the Supplementary Information , we also explore how the kinetics of this system can be modelled, and present a system in which the roles of the two invaders have been effectively reversed ( Supplementary Note 6 ; Supplementary Figs 8 and 9 ). 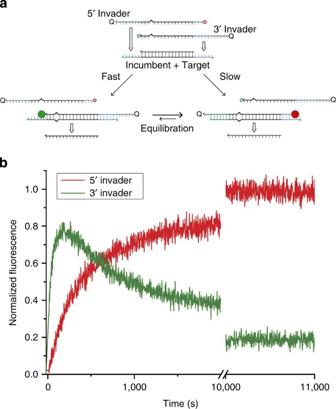Figure 4: A transient response controlled by an asymmetrically positioned mismatch. (a) Possible reactions in a system with two toeholds, two invaders and an asymmetric mismatch. The mismatch is proximal (4 nt) to the principal toehold for the 5′ invader and is thus a considerable impediment to displacement of the incumbent strand. For the 3′ invader, the mismatch is distal (13 nt), so the displacement rate is much faster. The 5′ invader, however, is complementary to three bases in the 3′ invader’s toehold domain and is thus strongly favoured thermodynamically, despite being at a kinetic disadvantage. (b) The hybridization of each invader can be tracked by measuring the intensities of spectrally separated fluorophores attached to their respective distal ends; in each case, fluorescence is initially quenched by the proximity of a quencher attached to the toehold end of the invader. In this experiment, 10 nM of each invading strand competed for an equimolar concentration of target initially bound to incumbent. Figure 4: A transient response controlled by an asymmetrically positioned mismatch. ( a ) Possible reactions in a system with two toeholds, two invaders and an asymmetric mismatch. The mismatch is proximal (4 nt) to the principal toehold for the 5′ invader and is thus a considerable impediment to displacement of the incumbent strand. For the 3′ invader, the mismatch is distal (13 nt), so the displacement rate is much faster. The 5′ invader, however, is complementary to three bases in the 3′ invader’s toehold domain and is thus strongly favoured thermodynamically, despite being at a kinetic disadvantage. ( b ) The hybridization of each invader can be tracked by measuring the intensities of spectrally separated fluorophores attached to their respective distal ends; in each case, fluorescence is initially quenched by the proximity of a quencher attached to the toehold end of the invader. In this experiment, 10 nM of each invading strand competed for an equimolar concentration of target initially bound to incumbent. Full size image The kinetic behaviour of the 3′ invader observed in this system (green trace in Fig. 4b ) is very similar to the current response of an overdamped linear resistor–inductor–capacitor circuit, which can be used to provide pulsed discharges (for example, see ref. 35 ). Our DNA-based device could conceivably serve a similar purpose within a multi-component nucleic-acid reaction network, enabling transient provision of a specific invader–target complex or serving as a temporary storage device for the kinetically favoured invading strand. As switching from uptake to release occurs spontaneously, and the storage parameters are tuneable via toehold strengths and mismatch positions, the device could serve as a fully autonomous actuator for reactive processes or dynamic DNA devices. Similar dynamic behaviour could be achieved by other system architectures [36] , [37] : the use of mismatches to engineer reaction rates requires a minimal number of components, however, decreasing the probability of unwanted side and leak reactions. We have demonstrated that we can control the rate of DNA strand displacement by altering the energy landscape via the position of a single mismatch created in the invader–target duplex. In contrast to most previous kinetic control methods, the rate constant for strand displacement can be tuned over three orders of magnitude without significantly changing the reaction free energy. Only small changes are necessary: the reaction system can be tuned over the full range by changing the identity of only two bases in the invading displacement domain. We note that toehold exchange [18] , a strand-exchange reaction in which the incumbent strand has its own toehold on the target strand that extends beyond the end of the displacement domain, has an energy landscape similar to that with a mismatch near the end of the displacement domain. This system also has the potential to allow kinetic control with approximately constant if both toeholds are adjusted such that the difference between toehold binding strengths is approximately constant [18] . Toehold exchange has proven to be an extremely effective mechanism for engineering fast reactions that are not strongly thermodynamically driven, and is also a basic primitive for nucleic-acid-based computational circuitry [37] . However, toehold-exchange systems that operate in the well-characterized second-order limit require short invading toeholds if kinetic control of the forward reaction is to be implemented while maintaining an intrinsic thermodynamic drive towards the product. Shorter toeholds reduce the potential for discrimination between invading strands on the basis of their toeholds, and are potentially more vulnerable to leak reactions. Toeholds are also frequently subject to constraints imposed by other parts of a reaction system: changing toeholds to tune reaction rates disrupts the modular design of strand-displacement networks and requires significant strand redesign. The repositioning of a mismatch in a displacement domain, in contrast, leaves all toeholds unaffected and can be implemented by the redesign of a single strand (the invader). We have also demonstrated that the decoupling of kinetics and thermodynamics provides useful engineering design capability by creating a simple DNA device that displays complex dynamic behaviour. The creation of mismatched base pairs has been used to slow strand displacement, but the marked and systematic dependence of displacement rate on mismatch location has not previously been demonstrated because mismatches were far from the distal end of the displacement domain [23] , [24] , [26] , [27] , the displacement domain was capped by an incumbent toehold [22] , [25] or reaction kinetics were not measured [21] . Our findings are likely to make an important contribution to the design of strand-displacement-based nucleic-acid probes [21] , [22] , [24] , [26] : methods based on measurements of reaction rates will struggle to detect mismatches between probe and target base sequences at the distal end of a displacement domain, whereas equilibrium-based approaches involving toehold exchange are much less sensitive to the position of a defect in the probe [21] , [22] . This study will also contribute to the design of nanoscale systems and devices which necessarily include mismatches, for example, to mask restriction enzyme recognition sites [10] or to reduce leak reactions in catalytic DNA circuits [28] . By calculating energy landscapes for strand displacement with single-nucleotide resolution, we are able to provide a qualitative explanation of the observed behaviour and near-quantitative prediction of relative reaction rates. The ability of oxDNA, a coarse-grained model with no free parameters, to provide insight into this reaction mechanism is an encouraging step towards the rational design and optimization of DNA nanotechnology. DNA oligonucleotides DNA oligonucleotide sequences were designed using NUPACK [33] . Temperature and salt concentrations were chosen to represent reaction conditions; the dangles option was set to ‘all’. Strands were designed to minimize secondary structures. We imposed a further constraint that no base should be repeated >3 times consecutively. Sequences for all experiments are listed in Supplementary Tables 6–10 . DNA oligonucleotides were acquired from Integrated DNA Technologies. Unlabelled strands were supplied desalted; labelled strands were HPLC purified before shipping. According to the manufacturer, oligonucleotide purity for unpurified strands can be expected to exceed 0.99 n , where n is the number of nucleotides in the strand. Samples were resuspended in Milli-Q purified water to a concentration of 100 μM, using the manufacturer’s information on amount of oligo per tube. For representative strands, the stock concentration was confirmed with 260 nm absorbance measurements at room temperature, and conversion from optical density to concentration using extinction coefficients based on the nearest-neighbour model [38] . Fluorescent reporter strands were titrated against the complementary quencher strand. Samples were stored at 4 °C. We chose Cy3 and Cy5 as fluorescent labels for our experiments, with IowaBlack® FQ and IowaBlack RQ, respectively, serving as quenchers. Design rationale for the reporter system Use of a reporter complex to measure strand displacement greatly increases the range of systems that can be experimentally tested without the need to prepare any further labelled oligonucleotides. This reporter consists of two strands initially bound to each other, one labelled with a fluorophore, the other with a quencher. Due to the spatial proximity of fluorophore and quencher, the fluorescence is supressed. Free incumbent can displace the fluorescently labelled strand (incumbent bound to target can also displace the fluorescently labelled strand, but the rate of this reaction is negligible [18] ). Once incumbent has displaced the fluorescently labelled strand, the fluorophore is no longer quenched: the change in bulk fluorescence can be used to track the progress of the overall reaction. To make measurements made using this reporter complex as comparable to each other as possible, we devised a simple strategy to make the different target/incumbent/invader systems as thermodynamically similar as possible. We briefly describe this strategy below. The perfectly matched system is shown in Table 1 (an invader toehold of 7 bases is used for illustrative purpose, but any choice between 0 and 10 is possible). We decided to focus on a single mismatch, as it is one of the single-base mismatches with the greatest energetic penalty [34] and we thus expected it to yield the most obvious impacts on displacement kinetics. The target strand contains the sequence TCA at the beginning of the displacement domain. To introduce the mismatch two nucleotides from the invader toehold (mismatch position 2), we thus have to change just one base in the invading strand, as shown in Table 1 . To minimize the variation in the overall standard free-energy of formation of the invader–target and incumbent–target duplexes, the mismatch location was changed by displacing bases from in front of the mismatch motif to behind it. This change does not affect the overall base composition of the strands, only the base sequence. Table 1 A series of sequences illustrating how the mismatch was moved to different positions Full size table This method is only possible until mismatch position 10; beyond this, the GGTGAG domain in the incumbent could not be altered as it forms the toehold necessary to release the reporter. Instead, this domain provides for another mismatch (at position 14) and an equivalent mismatch (at position 12), which only require modifications in the invader strand sequence. These modifications are also shown in Table 1 . This method allows for the testing of many different positions of the same mismatch, while varying the free energy of the invader–target duplex by <−1 kcal mol −1 , and the overall free-energy change of reaction by <−1.2 kcal mol −1 , as estimated by NUPACK [33] . Fluorimetry experiments All fluorimetry experiments were performed at 23 °C in a Fluoromax-3 (JY Horiba) in buffer containing 50 mM NaCl, 10 mM MgCl 2 and 10 mM Tris balanced to a pH of 8.0 using HCl. Most experiments were conducted in Hellma Analytics cuvettes in a 1.5-ml volume. Five experiments presented in Supplementary Note 5 and Supplementary Fig. 7 were instead conducted in Starna cuvettes in a 0.15-ml volume (those listed with a concentration ≥50 nM in Supplementary Table 8 ). The cuvettes were covered with lids or mineral oil (Sigma Aldrich) during experiments to prevent sample evaporation. Excitation/emission wavelengths were 649 nm/664 nm and 548 nm/563 nm for Cy5 and Cy3, respectively. Slit widths were set to 1 nm/1 nm for two-toehold-device measurements, and 2 nm/2 nm for all others. Data points were acquired every 2.1 s (for fast reactions) to 60 s (for slow reactions) with an integration time of 2 s. With these parameters, significant photobleaching as well as crosstalk between the Cy3 and Cy5 channels could be avoided. The photodetector was operated within its linear range. For the experiments with reporter, incumbent–target duplex and invader were subsequently added to a cuvette containing a solution of reporter complex. For those experiments where the incumbent and target strand were directly labelled, the invader was added to a cuvette containing buffer solution of the labelled incumbent–target duplex. For the two-toehold experiments, incumbent–target duplex was added to a cuvette containing the two dual-labelled invaders. Before adding further reagents to the cuvettes, signals were allowed to stabilize for at least 300 s. The baseline signal was subtracted from subsequently recorded fluorescence intensities. Addition of reagents was always performed in the same fashion, such that the first data point was acquired ca. 10 s after addition. Sample mixing was achieved by rapidly pipetting the reagent solution. Cuvettes were cleaned by washing twice with 100% ethanol, five times with Milli-Q purified water and again twice with 100% ethanol. Outer cuvette surfaces were cleaned with lens-cleaning tissues soaked in 100% ethanol. Fluorimetry data were processed using OriginPro 8.5.1 and Matlab R2011b. Rate constant fitting procedure Assuming displacement complexes quickly resolve into products or reactants, and therefore that all reactions can be modelled as instantaneous, second-order processes, we have where I is the invader, T is the target, O the incumbent, R the reporter, Q the quencher and XY a duplex consisting of strands X and Y. These reactions are modelled by the differential equations where k and k rep are the second-order rate constants of the displacement of the incumbent by invader and the reporter by the incumbent, respectively. The determination of k rep is outlined further below. Three different methods to derive the rate constant k were tested. The time-dependent values of [ R ], the concentration of free reporter strand, can be inferred directly from the fluorimetry data: the intensity of reporter fluorescence is linearly dependent on [ R ]. These data are fitted for variables k and c (with k rep and initial concentrations as fixed inputs), with c being a scaling factor to convert concentration of R measured in arbitrary fluorescence units to moles per litre. Both in approach and implementation, we closely followed Zhang and Winfree [18] . Values for k plotted in Fig. 2d were obtained by this method. A separate set of differential equations and Matlab functions were used to perform a similar fitting routine on data measured with the two-toehold system ( Supplementary Note 6 ; Supplementary Fig. 8 ). In the limit in which the reporter reaction is much faster than the displacement of the incumbent by the invader, the above system of differential equations can be solved analytically to give where [ X ] 0 indicates the initial concentration of component X (to derive this result, we have used [ I ] 0 =[ TO ] 0 ). Fitting this analytical solution provides a second estimate of rate constant k . A third method to derive rate constants from estimates of the half-completion time t 1/2 was also explored. First, a scaling factor to convert fluorescence intensity to concentration of R measured in moles per litre was estimated from the average of two baseline-corrected saturation fluorescence intensities from displacement reactions performed with the non-mismatched 10-nt toehold invader. The resultant scaling factor was found to be closely equal to the mean of all scaling factors derived from the differential-equation-based method described above. With the aid of this scaling factor estimate, the first point in each experimental time series was identified in which the reaction had surpassed half-completion. t 1/2 was estimated by linear interpolation between this and the previous data point. Reaction rate constants were then determined using Second-order reaction rate constants derived using all three methods are plotted in Supplementary Fig. 10 . All methods show the same systematic dependence of reaction kinetics on mismatch position. Deviations are most pronounced for fast reactions, which is unsurprising as in this case the approximation of an infinitely fast reporter breaks down, resulting in an underestimate of the rate constant in the analytical fits and half-completion-time estimates. The agreement between methods for the slower reactions emphasizes the reliability of our modelling and fitting procedure. Reporter system characterization The rate constant k rep for reporter displacement by the unattached incumbent was measured for each incumbent. Incumbent (6.7 nM) was added to a cuvette containing a stoichiometric quantity of the reporter complex. Supplementary Fig. 11 shows the resulting change in fluorescence, which is very similar for each of the samples: we attribute minor differences to uncertainties in determining concentrations and pipetting errors. These curves were fitted to determine a k rep using the equation The mean of the resulting rate constants is k rep =(2.1±0.4) × 10 6 M −1 s −1 . The individually fitted rate constant for each incumbent was used in subsequent fits using the numerical, differential-equation approach to determine rate constants for strand displacement. Use of the mean value of k rep in all cases produced very similar results. OxDNA implementation We considered four strand-displacement systems, distinguished by the presence and location of a mismatch between the invader and target. The systems were designed to mimic those of the 5-nt toehold invader tested experimentally ( Supplementary Table 9 ), without a separate reporter complex. We shall refer to the systems as perfectly matched, proximal mismatch, central mismatch and distal mismatch. All simulations were performed at 25 °C. This is 2 °C higher than the temperature of the experimental system—the sensitivity of DNA to such temperature differences is much smaller than the effects we have measured in this work. Due to the large enthalpic barrier to duplex dissociation, it is these processes that are most affected by temperature changes [39] . From the known thermodynamics of oxDNA [29] we estimate that reducing the temperature by 2 °C would slow the dissociation of a 5-base-pair duplex by a factor of ~1.5, which would not qualitatively influence our results. Kinetic simulations were performed using a Langevin Dynamics algorithm [40] augmented with forward flux sampling (FFS) [41] , [42] . Both are discussed in detail in Supplementary Note 3 . In our simulations, we simplified the system by prohibiting interstrand base pairs that were not native to either the initial target/incumbent duplex or the final target/invader duplex. This was done to avoid the complication of misbonded metastable states that are difficult to deal with using forward flux sampling. Preliminary simulations without this restriction indicated that metastable misbonds between the invader and target could form, but would typically then dissociate rather than rearranging to a toehold-bound state via internal displacement, a mechanism discussed previously [43] . This is consistent with our observations in previous studies of strand displacement [19] , and our work on hybridization rates for non-repetitive sequences [43] , in which non-native base pairs were seen to contribute only a small amount to overall hybridization for non-repetitive sequences. For computational tractability, we have simulated systems in a relatively small volume, giving strand concentrations of ~100 μM. This is much higher than in the experiments, which were performed at ~10 nM. In oxDNA, all interactions are short-ranged and hence the strands behave ideally unless they come into contact. Thus the effect of dilution on the system is trivial: using a cell of twice the volume halves the rate of association. Dilution should not, however, affect the rate at which a complex of strands breaks up or undergoes a structural rearrangement. In our simulations, the three-stranded complex has a lifetime that is smaller than, but comparable to, typical binding times. Were we to dilute the system by a factor of over 1,000, however, resolution of the intermediate complex would be much faster than typical times required for binding. For comparison with experiments, we therefore neglect the actual time spent in the three-stranded intermediate complex when estimating the relative overall rates. Instead, we first estimate the rates of association of the toeholds of the target and invader by calculating the flux from a dissociated state to the toehold-bound state. We then multiply this rate by the probability that such a state eventually leads to successful displacement rather than detaching, ignoring the actual time taken to do this. Order parameters for FFS were based on the separation of strands and the degree of base-pairing between strands. To do this, it is useful to define ‘nearly formed base pairs’. For two bases to qualify as nearly formed, three conditions have to be fulfilled. (1) The separation of hydrogen-bonding sites must be ≤0.85 nm. (2) The hydrogen-bonding potential consists of a separation-dependent factor multiplied by a number of modulating angular factors: at most one of these factors that contributes multiplicatively to the hydrogen-bonding energy must be zero. (3) The calculated hydrogen-bonding interaction must be less negative (weaker) than −1.43 kcal mol −1 (typical hydrogen bonds have enthalpies of −3.6 kcal mol −1 in oxDNA). These conditions mean that the bases are close and fairly well aligned but not forming a strong base pair. Given these definitions, the order parameters used for FFS simulations are outlined in Supplementary Tables 11 and 12 . The lengths and numbers of simulations run, and the results for each stage, are presented in Supplementary Tables 2 and 3 . We used the same FFS setup to measure the rate at which toeholds formed in all four systems. For the perfectly matched and distal mismatch cases, brute force simulation initiated from the toehold-bound states proved sufficient to determine the probability of success from that point (this is just like adding an additional FFS interface). The proximal and central mismatch systems proved more challenging, however. In these cases, the toehold-bound state is a metastable intermediate with a low probability of progressing to complete displacement, making the success probability from this point difficult to estimate by brute force simulation. Instead, we performed a second stage of FFS initiated from the toehold-bound state to measure the fluxes for detachment and successful displacement explicitly, and then use these values to calculate the success probability. This procedure relies on the assumption that the system equilibrates within the metastable toehold-bound state prior to either completing displacement or detaching, which is reasonable given the free-energy barriers along both paths. The free-energy landscapes presented in Fig. 3 were obtained using Virtual Move Monte Carlo [44] augmented by umbrella sampling [45] (both described in Supplementary Note 3 ). Simulations were performed using a three-dimensional reaction coordinate, the first dimension being the number of target/incumbent base pairs, the second being the number target/invader base pairs and the third identifying whether the two duplexes were disrupted at the outside edges (allowing the umbrella potential to favour disruption of base pairs at the junction and thereby accelerate branch migration). In this case, bases were considered paired if their hydrogen-bonding energy was more negative than −0.6 kcal mol −1 . This value has previously been used to characterize base pairing in oxDNA [29] , and is ideal because base pairs with this interaction strength are rarely observed (pairs of bases usually have much lower energies if bound). We note that this value is distinct from that used to define the reaction coordinate for FFS: this is because the two reaction coordinates perform different functions. For umbrella sampling, we want a criterion that neatly divides bound and unbound states. For FFS, we want a threshold that indicates that the formation of a strong base pair is very likely once the threshold is reached. Sampling simulations were performed using the biasing weights given in Supplementary Tables 13–16 . For each of the four systems, four independent simulations were run for 4 × 10 10 attempted Virtual Move Monte Carlo steps after an initialization period of 4 × 10 8 steps. Estimated errors based on these four independent simulations are <0.25 RT for the states that lie along the pathway in Fig. 3 . The results presented in the main text project the three-dimensional order parameter onto a two-dimensional representation involving the number of target/incumbent base pairs and the number of target/invader base pairs. How to cite this article: Machinek, R. R. F. et al. Programmable energy landscapes for kinetic control of DNA strand displacement. Nat. Commun. 5:5324 doi: 10.1038/ncomms6324 (2014).